Odour concentration-dependent olfactory preference change inC. elegans The same odorant can induce attractive or repulsive responses depending on its concentration in various animals including humans. However, little is understood about the neuronal basis of this behavioural phenomenon. Here we show that Caenorhabditis elegans avoids high concentrations of odorants that are attractive at low concentrations. Behavioural analyses and computer simulation reveal that the odour concentration-dependent behaviour is primarily generated by klinokinesis, a behavioural strategy in C. elegans . Genetic analyses and lesion experiments show that distinct combinations of sensory neurons function at different concentrations of the odorant; AWC and ASH sensory neurons have critical roles for attraction to or avoidance of the odorant, respectively. Moreover, we found that AWC neurons respond to only lower concentrations of the odorant, whereas ASH neurons respond to only higher concentrations of odorant. Hence, our study suggests that odour concentration coding in C. elegans mostly conforms to the labelled-line principle where distinct neurons respond to distinct stimuli. Animals possess an ability to detect a vast number of odorants, and show olfactory preference towards most odorants. It is empirically known that olfactory preference to the same odorant changes depending on the odorant concentration in some organisms including humans [1] , [2] , [3] . For example, an odorant indole included in jasmines and feces has a pleasant and floral smell at low concentrations, but is putrid when concentrated [3] . However, how information of the odour concentration is encoded in a neural network and how changes of odour concentrations lead to an olfactory preference switch are still poorly understood. The olfactory preference change depending on odour concentrations can be examined in detail in the nematode C. elegans , because all neurons and their entire connectivity pattern have been described [4] . C. elegans can detect a variety of volatile odorants and show chemotaxis to them. It has been reported that two behavioural strategies are used in attraction behaviour towards an attractive odour [5] , [6] . One is klinokinesis in which worms change the frequency of turning by sensing the odour gradient. The other is klinotaxis in which worms regulate curving rate bias by detecting the spatial odour gradient. The innate preference of C. elegans is exclusively determined by a labelled-line principle. The labelled-line theory suggests that stimuli of a particular given quality are encoded by cells that preferentially respond to that stimulus [7] . In C. elegans , dedicated sensory neurons are linked to specific behaviours such as attraction or avoidance; AWA and AWC olfactory neurons mediate the responses to attractive odorants, whereas sensory neurons called AWB, ASH and ADL mediate the responses to repellents [8] , [9] , [10] . However, the olfactory preference switch dependent on odour concentrations in C. elegans has not been well characterized. Here we show that olfactory preference of C. elegans also changes depending on the concentration of various odorants. The behavioural change from attraction to avoidance towards an odorant dependent on its concentration is mainly generated by klinokinesis. Laser ablation and genetic analyses reveal that distinct groups of sensory neurons are required for the attraction to and avoidance of an odorant at different concentrations. Moreover, calcium imaging shows that their neuronal responses to the odorant change depending on its concentration. Our results indicate that the odour concentration information in C. elegans is modulated at the sensory neuron level and is mostly based on the labelled-line theory. Odour concentration-dependent preference shift in C. elegans The nematode C. elegans is attracted to or repelled by a variety of volatile odorants, which are usually tested at low concentrations. For example, isoamyl alcohol, benzaldehyde, pentanedione, trimethylthiazole and diacetyl are known attractants [8] , while octanol and nonanone are repellents [9] . To examine whether the odour concentration-dependent preference change is also observed in C. elegans , we analysed its chemotaxis to attractive odorants when odorant concentrations were varied. At lower concentrations, worms showed attraction to the odorants as previously reported [8] ( Fig. 1a,b ). However, at higher concentrations, strong aversion was induced ( Fig. 1b ). These dose-dependent behavioural changes were observed in chemotaxis to all odorants tested ( Fig. 1b ). Higher concentrations of odorants placed on the lids of plates also induced avoidance behaviour, suggesting that this behaviour is not due to high osmolarity ( Fig. 1c ). These results indicate that the odorant preference of C. elegans alters depending on the concentration of various odorants, consistent with the previous reports that high concentrations of several odorants caused avoidance behaviour [8] , [11] , [12] . Because of the abundant knowledge about isoamyl alcohol based on laser ablation experiments, calcium imaging experiments and others, we focused on isoamyl alcohol in this study [8] , [13] . 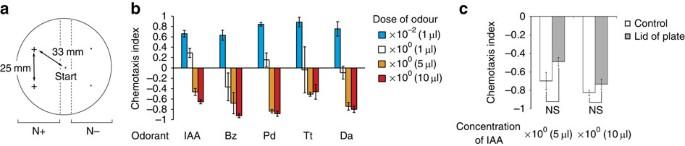Figure 1: Olfactory preference changes depending on the odour concentration inC. elegans. (a) A plate format that was mainly used in population chemotaxis assays unless otherwise indicated. Odorants were spotted on two points (plus marks) at one end of the assay plates, and sodium azide was spotted on two points at both ends of the plates. Animals were placed on the centre of the plate. After 1 h, the number of animals in each area (N+ and N−) was counted. Chemotaxis index=[(N+)−(N−)]/[(N+)+(N−)]. (b) Dose-dependent behavioural changes of wild-type animals to various odorants. IAA; isoamyl alcohol (N=8–9), Bz; benzaldehyde (N=8), Pd; pentanedione (N=7), Tt; trimetylthiazole (N=3), Da; diacetyl (N=10). (c) Responses of wild-type animals to higher concentrations of isoamyl alcohol when the odorant was spotted on plates (Control), or on the lids of plates (lid of plate);N=5. Student'st-test did not show significant difference (P>0.05). NS, not significant. Error bars represent s.e.m (b,c). Figure 1: Olfactory preference changes depending on the odour concentration in C. elegans . ( a ) A plate format that was mainly used in population chemotaxis assays unless otherwise indicated. Odorants were spotted on two points (plus marks) at one end of the assay plates, and sodium azide was spotted on two points at both ends of the plates. Animals were placed on the centre of the plate. After 1 h, the number of animals in each area (N+ and N−) was counted. Chemotaxis index=[(N+)−(N−)]/[(N+)+(N−)]. ( b ) Dose-dependent behavioural changes of wild-type animals to various odorants. IAA; isoamyl alcohol ( N =8–9), Bz; benzaldehyde ( N =8), Pd; pentanedione ( N =7), Tt; trimetylthiazole ( N =3), Da; diacetyl ( N =10). ( c ) Responses of wild-type animals to higher concentrations of isoamyl alcohol when the odorant was spotted on plates (Control), or on the lids of plates (lid of plate); N =5. Student's t -test did not show significant difference ( P >0.05). NS, not significant. Error bars represent s.e.m ( b , c ). Full size image To analyse how the animal's preference for an odorant changes depending on its concentration, we used a multiworm tracking system (Methods). In a gradient of lower concentrations of isoamyl alcohol, animals are constantly attracted to the odorant ( Fig. 2a ). However, in a gradient of higher concentrations of the odorant, animals showed initial attraction (until 600 s) then subsequent avoidance ( Fig. 2b–d, real worms). The behavioural switch from attraction to avoidance could be caused either by the animals' odour adaptation (olfactory plasticity) [14] or by a gradual increase of odorant concentration due to diffusion of the odorant. To distinguish between these possibilities, we observed avoidance behaviour of adaptation (plasticity)-deficient mutants [15] , [16] , [17] in the presence of higher concentrations of isoamyl alcohol ( Fig. 2e ). As these mutants did not show significant defects ( Fig. 2f ), we conclude that the increase of the odour concentration caused by diffusion is the major cause of the switch from attraction to avoidance. 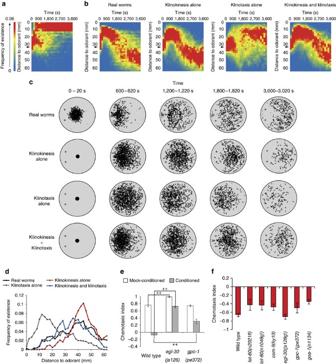Figure 2: Computer simulation analyses of avoidance behaviour towards a higher concentration of isoamyl alcohol. (a) The existence frequency at each distance to 1 μl of 10−2diluted isoamyl alcohol of wild-type animals;N=11 assays. (b) The existence frequency at each distance to 5 μl of undiluted isoamyl alcohol of wild-type animals (real worms), and computer-simulated animals with klinokinesis alone, klinotaxis alone and both mechanisms. Real worms,N=approximately 1,000 animals (nine assays); simulated animals,N=1,000 animals. Blue and red colours indicate the low and the high frequency of existence, respectively, of the animals in each region at the time indicated (a,b). Black triangles indicate start positions of animals. (c) Tracks of wild-type animals (real worms) and simulated animals with klinokinesis alone, klinotaxis alone and both mechanisms during chemotaxis to 5 μl of undiluted isoamyl alcohol. The odorant was spotted on two plus marks. Time interval is 20 s. All simulated animals started from the centre of the agar plate. Real worms,N=approximately 1,000 animals (nine assays); simulated animals,N=1,000 animals. (d) The existence frequency of real worms and simulated animals at 2,850 to 3,000 s during chemotaxis to 5 μl of undiluted isoamyl alcohol. Real worms,N=approximately 1,000; simulated animals,N=1,000. (e) Olfactory adaptation to isomayl alcohol of wild-type animals and mutants ofegl-30(js126) andgpc-1(pe372);N=6. Significant differences from wild-type animals are indicated by ++ (P<0.01, Dunnett's test). (f) Responses of wild-type animals and mutants oflet-60(n2021lf),let-60(n1041gf),osm-9(ky10),egl-30(js126),gpc-1(pe372)andgoa-1(n1134)to 10 μl of undiluted isoamyl alcohol. These mutants did not show significant defects in avoidance of a higher concentration of isoamyl alcohol (P>0.05, Dunnett's test),N=6–8. Error bars represent the s.e.m. (e,f). Figure 2: Computer simulation analyses of avoidance behaviour towards a higher concentration of isoamyl alcohol. ( a ) The existence frequency at each distance to 1 μl of 10 −2 diluted isoamyl alcohol of wild-type animals; N =11 assays. ( b ) The existence frequency at each distance to 5 μl of undiluted isoamyl alcohol of wild-type animals (real worms), and computer-simulated animals with klinokinesis alone, klinotaxis alone and both mechanisms. Real worms, N =approximately 1,000 animals (nine assays); simulated animals, N =1,000 animals. Blue and red colours indicate the low and the high frequency of existence, respectively, of the animals in each region at the time indicated ( a , b ). Black triangles indicate start positions of animals. ( c ) Tracks of wild-type animals (real worms) and simulated animals with klinokinesis alone, klinotaxis alone and both mechanisms during chemotaxis to 5 μl of undiluted isoamyl alcohol. The odorant was spotted on two plus marks. Time interval is 20 s. All simulated animals started from the centre of the agar plate. Real worms, N =approximately 1,000 animals (nine assays); simulated animals, N =1,000 animals. ( d ) The existence frequency of real worms and simulated animals at 2,850 to 3,000 s during chemotaxis to 5 μl of undiluted isoamyl alcohol. Real worms, N =approximately 1,000; simulated animals, N =1,000. ( e ) Olfactory adaptation to isomayl alcohol of wild-type animals and mutants of egl-30 ( js126 ) and gpc-1 ( pe372 ); N =6. Significant differences from wild-type animals are indicated by ++ ( P <0.01, Dunnett's test). ( f ) Responses of wild-type animals and mutants of let-60(n2021lf) , let-60(n1041gf) , osm-9(ky10) , egl-30(js126) , gpc-1(pe372) and goa-1(n1134) to 10 μl of undiluted isoamyl alcohol. These mutants did not show significant defects in avoidance of a higher concentration of isoamyl alcohol ( P >0.05, Dunnett's test), N =6–8. Error bars represent the s.e.m. ( e , f ). Full size image Behavioural regulation by two behavioural strategies Previous studies have reported that C. elegans uses two behavioural strategies, klinokinesis and klinotaxis for attraction to water-soluble chemoattractants such as NaCl (refs 5 and 6 ; Fig. 3a,b ). In klinokinesis, also called the pirouette strategy, when the worm senses a decrease in the concentration of a favoured chemical, it then turns by a 'pirouette' behaviour and randomly chooses a new forward direction ( Fig. 3a ). In klinotaxis, also called the weathervane strategy, the worm responds to a spatial gradient of a favoured chemical by gradually curving towards the higher concentration ( Fig. 3b ). To investigate how odour concentration-dependent behaviour is generated, we observed klinokinesis and klinotaxis in gradients of lower or higher concentrations of isoamyl alcohol. In chemotaxis to a lower concentration of isoamyl alcohol, klinokinesis was used to drive attraction at all time points ( Fig. 3c ), and klinotaxis was also used in the direction towards the odorants after 1,500 s ( Fig. 3d ). Klinotaxis was not observed at the beginning of the assays probably due to insufficient diffusion of the odorant, because klinotaxis was detected from the start of experiments when odour sources were spotted closer to the animals ( Fig. 3e,f ). In chemotaxis to a higher concentration of isoamyl alcohol, klinokinesis was used to drive attraction until 300 s, and then acted in the opposite direction after 600 s ( Fig. 3c,g ), which is consistent with the behaviour observed in Fig. 2b (real worms). On the other hand, unexpectedly, klinotaxis was used in the direction to drive attraction to the odorant ( Fig. 3d,h ). These results indicate that the behavioural change depending on the odour concentration is mainly regulated by klinokinesis. 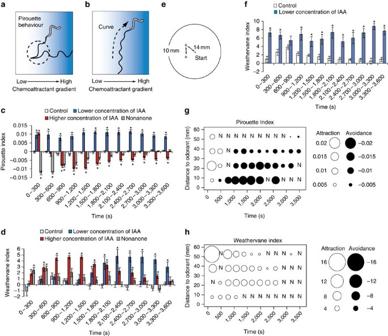Figure 3: Klinokinesis and klinotaxis mechanisms during chemotaxis to odour. (a,b) Schematic representations of klinokinesis (a) and klinotaxis (b). Blue shading indicates the concentration gradient of a chemoattractant. Dotted line circle indicates a pirouette behaviour composed of a reversal and omega-turn. (c,d) Klinokinesis (c) and klinotaxis (d) during chemotaxis to no gradient of an odorant (Control), a lower concentration of isoamyl alcohol (IAA; 1 μl of 10−2dilution), a higher concentration of isoamyl alcohol (5 μl of undilution) and nonanone (1 μl of 10−1dilution);N=8–10. (e) A plate format used to measure klinotaxis inFig. 3f. One μl each of an odorant was spotted on two plus marks closer to an animal compared with the normal chemotaxis plate shown inFig. 1a. (f) Klinotaxis of wild-type animals during chemotaxis to control (no gradient of an odorant) and a lower concentration of isoamyl alcohol (1 μl of 10−4dilution) when the odour was spotted closer to animals;N=9–10. Significant differences from the control are indicated by * (P<0.05, Dunnett's test;c,d,f). Error bars represent the s.e.m. (g,h) Klinokinesis (g) and klinotaxis (h) of wild-type animals during chemotaxis to 5 μl of undiluted isoamyl alcohol;N=9. The diameter of the circle at each position represents the value of the pirouette index (g) or the weathervane index (h), at the time and at the distance from an animal to an odour source. The interval of time and distance are 300 s and 15 mm, respectively. The sizes of circles indicate their values of indices. Closed and open circles indicate that each strategy operates to drive attraction and avoidance, respectively, towards an odorant. 'N' indicates that the values of indices are not significantly different from 0 by Student'st-test (P>0.05). Figure 3: Klinokinesis and klinotaxis mechanisms during chemotaxis to odour. ( a , b ) Schematic representations of klinokinesis ( a ) and klinotaxis ( b ). Blue shading indicates the concentration gradient of a chemoattractant. Dotted line circle indicates a pirouette behaviour composed of a reversal and omega-turn. ( c , d ) Klinokinesis ( c ) and klinotaxis ( d ) during chemotaxis to no gradient of an odorant (Control), a lower concentration of isoamyl alcohol (IAA; 1 μl of 10 −2 dilution), a higher concentration of isoamyl alcohol (5 μl of undilution) and nonanone (1 μl of 10 −1 dilution); N =8–10. ( e ) A plate format used to measure klinotaxis in Fig. 3f . One μl each of an odorant was spotted on two plus marks closer to an animal compared with the normal chemotaxis plate shown in Fig. 1a . ( f ) Klinotaxis of wild-type animals during chemotaxis to control (no gradient of an odorant) and a lower concentration of isoamyl alcohol (1 μl of 10 −4 dilution) when the odour was spotted closer to animals; N =9–10. Significant differences from the control are indicated by * ( P <0.05, Dunnett's test; c , d , f ). Error bars represent the s.e.m. ( g , h ) Klinokinesis ( g ) and klinotaxis ( h ) of wild-type animals during chemotaxis to 5 μl of undiluted isoamyl alcohol; N =9. The diameter of the circle at each position represents the value of the pirouette index ( g ) or the weathervane index ( h ), at the time and at the distance from an animal to an odour source. The interval of time and distance are 300 s and 15 mm, respectively. The sizes of circles indicate their values of indices. Closed and open circles indicate that each strategy operates to drive attraction and avoidance, respectively, towards an odorant. ' N ' indicates that the values of indices are not significantly different from 0 by Student's t -test ( P >0.05). Full size image To determine relative contributions of these opposite-directional behavioural strategies, we performed a computer simulation ( Supplementary Fig. S1 ). With klinokinesis alone, model animals showed initial attraction to the odorant followed by avoidance, similar to, but not identical to real worms ( Fig. 2b–d, klinokinesis alone). When klinotaxis alone was implemented, model animals showed only attraction behaviour to the odour ( Fig. 2b–d, klinotaxis alone). With both strategies at work, the behaviour of model animals looked like that of real worms ( Fig. 2b–d, klinokinesis and klinotaxis). These results indicate that klinokinesis has a major role in the avoidance of higher concentrations of isoamyl alcohol, while klinotaxis slightly weakens the avoidance by acting in the direction opposite to klinokinesis. To investigate how two behavioural mechanisms are also used in avoidance of a pure repellent, we observed the behaviour in the response to nonanone, which is an aversive odorant [9] . Different from the avoidance of higher concentrations of isoamyl alcohol, klinokinesis continuously drove avoidance while klinotaxis was hardly observed ( Fig. 3c,d ). The existence of higher concentrations of chemoattractants on an agar plate may be similar to the situation of simultaneous presence of a food and repellent in nature. If so, simultaneous use of opposite-directional strategies would prevent worms from moving too far away from the food source. A G α ODR-3 mediates bidirectional behavioural responses We then asked what molecules mediate the behaviour. We focused on the G-protein α -subunits, because they have major roles in the olfactory signalling pathway in sensory neurons. C. elegans contains 20 G α genes in its genomic sequence [18] . Among them, ODR-3 and GPA-3 are known to be involved in the response to lower concentrations of isoamyl alcohol [19] . In chemotaxis to higher concentrations of isoamyl alcohol, odr-3 mutants showed a severe defect, but other G α mutants including gpa-3 did not show significant defects ( Fig. 4a–c ). Moreover, odr-3 gpa-3 double mutants did not show additive defects compared with odr-3 single mutants ( Fig. 4a ). These results indicate that mainly ODR-3 functions in the response to both lower and higher concentrations of isoamyl alcohol, causing attractive and repulsive behaviours, respectively. The odr-3 gpa-3 mutants showed attraction to higher concentrations of isoamyl alcohol ( Fig. 4a ), indicating that other G α probably works in sensing undiluted isoamyl alcohol and driving attractive behaviour. ODR-3 is also known to mediate attraction to various odorants such as benzaldehyde and diacetyl at lower concentrations [20] , and initial attraction to but not subsequent avoidance of undiluted benzaldehyde [21] . In contrast to isoamyl alcohol, ODR-3 is not involved in avoidance of higher concentrations of benzaldehyde or diacetyl, as previously reported [14] ( Fig. 4d ). 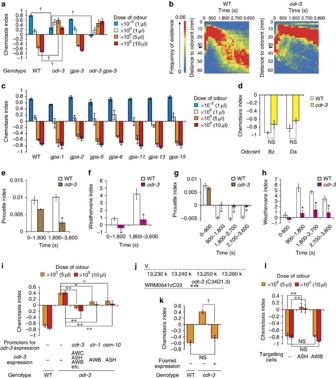Figure 4: G-proteinα-subunit ODR-3 mediates the response to isoamyl alcohol depending on its concentration. (a) Dose-dependent responses to isoamyl alcohol of wild-type animals and mutants ofodr-3,gpa-3andodr-3 gpa-3;N=5–7. (b) The existence frequency of wild-type animals (N=9) and theodr-3mutants (N=7) during chemotaxis to 5 μl of undiluted isoamyl alcohol. Black triangles indicate the start position of animals. (c) Dose-dependent behaviour of mutants of Gαproteins to isoamyl alcohol;N≥4. (d) Responses of theodr-3mutants to 5 μl of undiluted benzaldehyde (Bz;N=6) and diacetyl (Da;N=6). (e,f) Effects ofodr-3mutation to klinokinesis (e) and klinotaxis (f) during chemotaxis to a lower concentration of isoamyl alcohol (1 μl of 10−2dilution). Wild type,N=11;odr-3,N=8. (g,h) Effects ofodr-3mutation to klinokinesis (g) and klinotaxis (h) during chemotaxis to a higher concentration of isoamyl alcohol (5 μl of undiluted odour). Wild type,N=11;odr-3,N=7. (i) Responses to undiluted isoamyl alcohol of theodr-3mutants expressingodr-3cDNA under various promoters;N=8–10. (j) Genomic positions ofodr-3and a fosmid (WRM0641cC03) containing theodr-3gene. (k) Responses to a higher concentration of isoamyl alcohol (5 μl of undiluted odour) of theodr-3mutants expressing the fosmid (WRM0641cC03);N=9. (l) Responses to higher concentrations of isoamyl alcohol of wild-type animals with cell-specific knockdown ofodr-3;N=5. Error bars represent the s.e.m. (a,c–i,k,l). Significant differences are indicated by † (P<0.01) using Tukey's test, ++ (P<0.01), + (P<0.05) by Dunnett's test and * (P<0.05) by Student'st-test. NS, not significant; WT, wild type. Figure 4: G-protein α -subunit ODR-3 mediates the response to isoamyl alcohol depending on its concentration. ( a ) Dose-dependent responses to isoamyl alcohol of wild-type animals and mutants of odr-3 , gpa-3 and odr-3 gpa-3 ; N =5–7. ( b ) The existence frequency of wild-type animals ( N =9) and the odr-3 mutants ( N =7) during chemotaxis to 5 μl of undiluted isoamyl alcohol. Black triangles indicate the start position of animals. ( c ) Dose-dependent behaviour of mutants of G α proteins to isoamyl alcohol; N ≥4. ( d ) Responses of the odr-3 mutants to 5 μl of undiluted benzaldehyde (Bz; N =6) and diacetyl (Da; N =6). ( e , f ) Effects of odr-3 mutation to klinokinesis ( e ) and klinotaxis ( f ) during chemotaxis to a lower concentration of isoamyl alcohol (1 μl of 10 −2 dilution). Wild type, N =11; odr-3 , N =8. ( g , h ) Effects of odr-3 mutation to klinokinesis ( g ) and klinotaxis ( h ) during chemotaxis to a higher concentration of isoamyl alcohol (5 μl of undiluted odour). Wild type, N =11; odr-3 , N =7. ( i ) Responses to undiluted isoamyl alcohol of the odr-3 mutants expressing odr-3 cDNA under various promoters; N =8–10. ( j ) Genomic positions of odr-3 and a fosmid (WRM0641cC03) containing the odr-3 gene. ( k ) Responses to a higher concentration of isoamyl alcohol (5 μl of undiluted odour) of the odr-3 mutants expressing the fosmid (WRM0641cC03); N =9. ( l ) Responses to higher concentrations of isoamyl alcohol of wild-type animals with cell-specific knockdown of odr-3 ; N =5. Error bars represent the s.e.m. ( a , c – i , k , l ). Significant differences are indicated by † ( P <0.01) using Tukey's test, ++ ( P <0.01), + ( P <0.05) by Dunnett's test and * ( P <0.05) by Student's t -test. NS, not significant; WT, wild type. Full size image We next examined whether ODR-3 transmits sensory information used in the two behavioural strategies during chemotaxis to isoamyl alcohol at the lower and higher concentrations. In a gradient of lower concentrations of isoamyl alcohol, the odr-3 mutants were defective in klinokinesis after 1,800 s and klinotaxis at all times ( Fig. 4e,f ). Normal klinokinesis until 1,800 s may be due to functions of other G proteins such as GPA-3. Also in the gradient of higher concentrations of isoamyl alcohol, the odr-3 mutants showed considerable defects in klinokinesis to drive avoidance after 900 s and klinotaxis used in the direction towards the odorants after 900 s ( Fig. 4g,h ). These results indicate that ODR-3 regulates both klinokinesis and klinotaxis during attraction and avoidance, but not klinokinesis for initial attraction to the odorant. To determine the neurons in which ODR-3 functions to control avoidance of higher concentrations of isoamyl alcohol, we next performed cell-specific rescue and knockdown experiments by using various promoters. Expression of odr-3 cDNA from its own promoter rescued the avoidance defects of the odr-3 mutants ( Fig. 4i ). ODR-3 was previously reported to be expressed in five pairs of sensory neurons, AWA, AWB, AWC, ASH and ADF [20] . Among these neurons, AWB and ASH sensory neurons are known to mediate avoidance of volatile odorants [9] , [10] , [11] , [12] . Avoidance defects of the odr-3 mutants were rescued by either AWB- or ASH-specific expression of odr-3 cDNA ( Fig. 4i ). Because the fosmid containing the odr-3 gene fully rescued the avoidance defects of the odr-3 mutants, partial rescues by the odr-3 promoter may indicate that ODR-3 also functions in neurons other than those in which the 2.7-kb odr-3 promoter region drives expression ( Fig. 4j,k ) [20] . ADL sensory neurons might be candidates, because of previous reports that ADL are required for the avoidance of repellents [9] , [10] , [22] . Different from the results of cell-specific rescue experiments, the avoidance of isoamyl alcohol in wild-type animals was impaired by knockdown of odr-3 in ASH, but not in AWB neurons ( Fig. 4l ). The cause of difference between the rescue and knockdown experiments is discussed later. These behavioural-genetic analyses of odr-3 suggest that ODR-3 functions mainly in ASH sensory neurons to regulate avoidance of higher concentrations of isoamyl alcohol, supported by previous studies of the avoidance of water-soluble repellents [23] , [24] . It was previously suggested that ODR-3 mediates attraction to diluted isoamyl alcohol in AWC olfactory neurons [19] . Therefore, we propose that functions of ODR-3 in different sensory neurons mediate different behaviours, attraction or avoidance, in the response to isoamyl alcohol. Neural circuits for odour concentration-dependent behaviours Our above analyses demonstrate that different sets of sensory neurons are used for the response to lower and higher concentrations of isoamyl alcohol. To identify neural circuits regulating avoidance of higher concentrations of isoamyl alcohol, we killed candidate neurons using a laser microbeam, and observed the behavioural responses of the operated animals by manually recording their tracks ( Fig. 5a ). 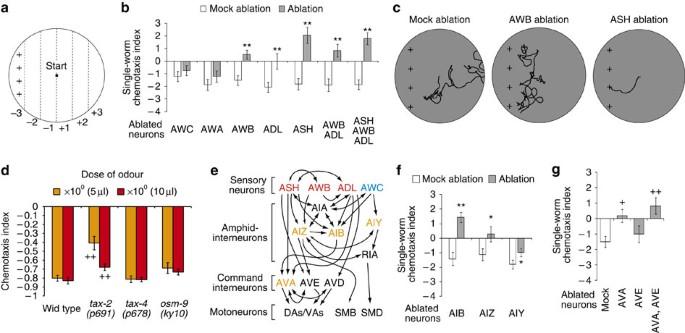Figure 5: Neural circuits regulating behaviour to higher concentrations of isoamyl alcohol. (a) A plate format used in single-worm chemotaxis assays of laser-ablated animals. Five μl each of undiluted isoamyl alcohol was spotted at four plus marks. An ablated animal was placed on the centre of the plate. The scores from −3 to +3 assigned to each sector are indicated. The single-worm chemotaxis index was calculated based on the sum of scores of the sectors in which a worm had travelled during 1 h. (b) Reponses to a higher concentration of isoamyl alcohol (5 μl of undilution) of animals with sensory neurons ablated. (c) Representative tracks of an individual animal with mock, AWB or ASH ablation. Five μl each of undiluted isoamyl alcohol was spotted on four plus marks. (d) Responses oftax-2,tax-4andosm-9mutants to higher concentrations of isoamyl alcohol. It was reported that the function of AWB sensory neurons is defective in mutants oftax-2ortax-4encoding a CNG channel, and that the function of ASH sensory neurons is defective in mutants ofosm-9encoding a TRP channel9,38. Thetax-2mutants showed a weak defect in the avoidance of isoamyl alcohol, indicating that AWB are involved in the avoidance of isoamyl alcohol at higher concentrations;N=6–7. (e) Diagrams of synaptic wiring including neurons tested in this study. Blue and red colours indicate sensory neurons mediating attraction to lower concentrations of isoamyl alcohol and avoidance of higher concentrations of isoamyl alcohol, respectively. Orange indicates interneurons involved in avoidance of higher concentrations of isoamyl alcohol. (f,g) Reponses to a higher concentration of isoamyl alcohol (5 μl of undilution) of animals with ablation of interneurons (f) or command interneurons (g). Error bars represent the s.e.m. (b,d,f,g). Significant differences from mock-ablated animals (b,f,g) or wild-type animals (d) are indicated by ** (P<0.01), * (P<0.05) using Student'st-test, and ++ (P<0.01), + (P<0.05) by Dunnett's test. Mock-ablated animals,N=24–64; ablated animals,N=16–52 (b,f,g). Figure 5: Neural circuits regulating behaviour to higher concentrations of isoamyl alcohol. ( a ) A plate format used in single-worm chemotaxis assays of laser-ablated animals. Five μl each of undiluted isoamyl alcohol was spotted at four plus marks. An ablated animal was placed on the centre of the plate. The scores from −3 to +3 assigned to each sector are indicated. The single-worm chemotaxis index was calculated based on the sum of scores of the sectors in which a worm had travelled during 1 h. ( b ) Reponses to a higher concentration of isoamyl alcohol (5 μl of undilution) of animals with sensory neurons ablated. ( c ) Representative tracks of an individual animal with mock, AWB or ASH ablation. Five μl each of undiluted isoamyl alcohol was spotted on four plus marks. ( d ) Responses of tax-2 , tax-4 and osm-9 mutants to higher concentrations of isoamyl alcohol. It was reported that the function of AWB sensory neurons is defective in mutants of tax-2 or tax-4 encoding a CNG channel, and that the function of ASH sensory neurons is defective in mutants of osm-9 encoding a TRP channel [9] , [38] . The tax-2 mutants showed a weak defect in the avoidance of isoamyl alcohol, indicating that AWB are involved in the avoidance of isoamyl alcohol at higher concentrations; N =6–7. ( e ) Diagrams of synaptic wiring including neurons tested in this study. Blue and red colours indicate sensory neurons mediating attraction to lower concentrations of isoamyl alcohol and avoidance of higher concentrations of isoamyl alcohol, respectively. Orange indicates interneurons involved in avoidance of higher concentrations of isoamyl alcohol. ( f , g ) Reponses to a higher concentration of isoamyl alcohol (5 μl of undilution) of animals with ablation of interneurons ( f ) or command interneurons ( g ). Error bars represent the s.e.m. ( b , d , f , g ). Significant differences from mock-ablated animals ( b , f , g ) or wild-type animals ( d ) are indicated by ** ( P <0.01), * ( P <0.05) using Student's t -test, and ++ ( P <0.01), + ( P <0.05) by Dunnett's test. Mock-ablated animals, N =24–64; ablated animals, N =16–52 ( b , f , g ). Full size image We first tried to identify which sensory neurons are required for the response to isoamyl alcohol at higher concentrations. Killing AWC, which are known to mediate attraction to lower concentrations of isoamyl alcohol, had no effect ( Fig. 5b ). Killing AWA, another class of attractant-sensing olfactory neurons [8] , also caused no defect ( Fig. 5b ). These results indicate that AWC and AWA are not involved in the response to higher concentrations of isoamyl alcohol. To determine which sensory neurons mediate avoidance of isoamyl alcohol, we examined the involvement of AWB and ADL neurons which were previously reported to be required for avoidance of repellents and higher concentrations of benzaldehyde [9] , [10] , [12] , [21] , [22] . AWB-ablated animals showed defects in avoidance of isoamyl alcohol at a higher concentration ( Fig. 5b ) and some animals showed initial attraction but no subsequent avoidance ( Fig. 5c ). This result is consistent with the defective phenotype in the response to higher concentrations of isoamyl alcohol of tax-2 mutants, which are known to lack functions of AWB [9] ( Fig. 5d ). ADL ablation decreased the avoidance just like killing AWB ( Fig. 5b ). Next, we tested the involvement of ASH neurons, in which ODR-3 functions mainly during isoamyl alcohol avoidance. Killing ASH remarkably diminished avoidance behaviour ( Fig. 5b ). Some ASH-ablated animals completely failed to avoid a higher concentration of isoamyl alcohol and died after touching the undiluted odorant ( Fig. 5c ). An AWB–ADL double ablation had no additive effect compared with AWB or ADL ablation alone, and an ASH–AWB–ADL triple ablation resembled an ASH ablation alone ( Fig. 5b ). These results indicate that ASH has major roles, and AWB and ADL have minor roles in mediating the animal's avoidance of higher concentrations of isoamyl alcohol. Taken together, we conclude that changes in the combination of sensory neurons underlie the worm's concentration-dependent olfactory preferences ( Fig. 5e ). We next examined the contribution of interneurons, which receive synaptic inputs from the above-mentioned sensory neurons regulating chemotaxis to higher concentrations of isoamyl alcohol ( Fig. 5e ). Previous reports suggested that AWC sensory neurons and downstream interneurons AIB and AIY regulate chemotaxis to lower concentrations of isoamyl alcohol [8] , [13] . On the basis of the neural wiring [4] , AIB interneurons receive synaptic inputs from ASH and ADL sensory neurons as well. Killing AIB decreased avoidance and instead caused attraction to isoamyl alcohol ( Fig. 5f ), suggesting that AIB interneurons have a major role for regulating avoidance of higher concentrations of isoamyl alcohol. Killing AIZ interneurons, which have synaptic inputs from ASH and AWB, also decreased avoidance behaviour ( Fig. 5f ). AIY are synaptically connected to AWC sensory neurons and AIZ interneurons, and AIY ablation caused a slight but significant defect in avoidance of isoamyl alcohol ( Fig. 5f ). These results indicate that AIB, AIZ and AIY interneurons are involved in mediating avoidance of higher concentrations of isoamyl alcohol and that the interneuron network that regulates the behavioural responses of C. elegans to higher concentrations of odorants partially overlaps with that regulating the response to lower concentrations of odorants [13] . ASH and ADL neurons also directly synapse onto AVA and/or AVE command interneurons, which drive backward locomotion [25] . Killing AVA considerably affected the avoidance of isoamyl alcohol, but killing AVE did not ( Fig. 5g ). Furthermore, the effect of AVA–AVE double ablation was identical to that of AVA ablation alone ( Fig. 5g ). These results indicate that AVA regulate avoidance of isoamyl alcohol, probably by controlling the backward locomotion, which could trigger a pirouette behaviour. Neural responses change depending on odour concentrations The results of our lesion experiments demonstrated that the behavioural change towards isoamyl alcohol depending on its concentration is mediated by different combinations of participating sensory neurons. Thus, we next investigated whether AWC, ASH and AWB sensory neurons respond to isoamyl alcohol, and if they responded, we tested whether their responses differ depending on the odour concentration. We monitored the responses of these neurons to isoamyl alcohol by calcium imaging using GCaMP [26] , [27] . A pair of AWC sensory neurons called AWC ON and AWC OFF are specified by asymmetric expression of odorant receptors [28] , and it was reported that both AWC ON and AWC OFF were activated by the removal of isoamyl alcohol [13] . We observed increases in AWC ON calcium ion levels on odour removal and considerable decreases on odour addition at 10 −4 and 10 −6 dilutions ( Fig. 6a,b ), consistent with the previous study [13] . On the other hand, we found that AWC ON did not respond to isoamyl alcohol at 10 −2 dilution ( Fig. 6a,b ). Because AWC ON responded normally to isoamyl alcohol at 10 −4 dilution after application of the odorant at 10 −2 dilution, addition of 10 −2 diluted odorant does not cause obvious damage to the AWC ON neuron ( Supplementary Fig. S2a,b ). To test whether the disappearance of the response of AWC ON to isoamyl alcohol at 10 −2 dilution is caused by itself or by an effect of synaptically connected neurons, we monitored the responses of AWC ON in unc-13 mutants, which have a deficit in synaptic vesicle exocytosis [29] . AWC ON in the unc-13 mutants considerably responded to 10 −2 diluted isoamyl alcohol ( Fig. 6c,d ), revealing the possibility that the response of AWC ON to higher concentrations of the odorant is regulated by suppression effects from other neurons. These results indicate that AWC ON becomes less sensitive to isoamyl alcohol under the influence of synaptic suppression by other neurons as the concentration of the odorant increases above a certain threshold. 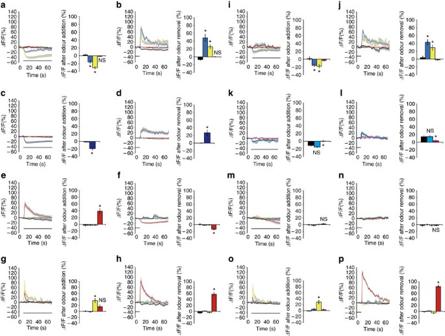Figure 6: Activity patterns of sensory neurons in the response to isoamyl alcohol change depending on its concentration. (a,b) GCaMP calcium responses of AWCONafter application (a) or removal (b) of no odour (Control, black) or different concentrations of isoamyl alcohol (10−6, blue; 10−4, yellow; 10−2, red) in wild-type animals;N=14–17. (c,d) Calcium responses of AWCONafter application (c) or removal (d) of 10−2diluted isoamyl alcohol in wild-type animals (red) andunc-13mutants (blue);N=17–26. (e,f) ASH calcium responses after application (e) or removal (f) of isoamyl alcohol in wild-type animals;N=9–21. (g,h) AWB calcium responses after application (g) or removal (h) of isoamyl alcohol in wild-type animals;N=10–25. (i,j) Calcium responses of AWCONinodr-3mutants after application (i) or removal (j) of isoamyl alcohol;N=9–20. Black, blue, yellow and red indicate no odorant (control), 10−6, 10−4and 10−2dilution of isoamyl alcohol, respectively (e–j). (k,l) Calcium responses of AWCONafter application (k) or removal (l) of 10−8diluted isoamyl alcohol in wild-type animals (black) and mutants ofodr-3(blue) andodr-3 gpa-3(magenta);N=16–22. (m–p) Calcium responses of ASH (m,n) and AWB (o,p) inodr-3mutants after application (m,o) or removal (n,p) of isoamyl alcohol;N=8–23. Black, blue, yellow and red indicate no odorant (control), 10−6, 10−4and 10−2dilution of isoamyl alcohol, respectively. Grey bars indicate presence of isoamyl alcohol, and the shaded regions around the curves represent the s.e.m. (a–p). Bar graphs show average fluorescence changes during the 10-s bins after odour addition or removal (seeMethods) and error bars represent the s.e.m. Significant differences from the control are indicated by * (P<0.05) using Dunnett's test. NS, not significant. Figure 6: Activity patterns of sensory neurons in the response to isoamyl alcohol change depending on its concentration. ( a , b ) GCaMP calcium responses of AWC ON after application ( a ) or removal ( b ) of no odour (Control, black) or different concentrations of isoamyl alcohol (10 −6 , blue; 10 −4 , yellow; 10 −2 , red) in wild-type animals; N =14–17. ( c , d ) Calcium responses of AWC ON after application ( c ) or removal ( d ) of 10 −2 diluted isoamyl alcohol in wild-type animals (red) and unc-13 mutants (blue); N =17–26. ( e , f ) ASH calcium responses after application ( e ) or removal ( f ) of isoamyl alcohol in wild-type animals; N =9–21. ( g , h ) AWB calcium responses after application ( g ) or removal ( h ) of isoamyl alcohol in wild-type animals; N =10–25. ( i , j ) Calcium responses of AWC ON in odr-3 mutants after application ( i ) or removal ( j ) of isoamyl alcohol; N =9–20. Black, blue, yellow and red indicate no odorant (control), 10 −6 , 10 −4 and 10 −2 dilution of isoamyl alcohol, respectively ( e – j ). ( k , l ) Calcium responses of AWC ON after application ( k ) or removal ( l ) of 10 −8 diluted isoamyl alcohol in wild-type animals (black) and mutants of odr-3 (blue) and odr-3 gpa-3 (magenta); N =16–22. ( m – p ) Calcium responses of ASH ( m , n ) and AWB ( o , p ) in odr-3 mutants after application ( m , o ) or removal ( n , p ) of isoamyl alcohol; N =8–23. Black, blue, yellow and red indicate no odorant (control), 10 −6 , 10 −4 and 10 −2 dilution of isoamyl alcohol, respectively. Grey bars indicate presence of isoamyl alcohol, and the shaded regions around the curves represent the s.e.m. ( a – p ). Bar graphs show average fluorescence changes during the 10-s bins after odour addition or removal (see Methods ) and error bars represent the s.e.m. Significant differences from the control are indicated by * ( P <0.05) using Dunnett's test. NS, not significant. Full size image We next monitored the activity of ASH sensory neurons that have major roles for avoidance of isoamyl alcohol at higher concentrations. A previous study showed that addition of a variety of noxious stimuli evokes increases in ASH calcium ion levels [30] . In contrast to AWC ON maximal increases were observed at 10 −2 dilution, while considerable increases were not detected at 10 −4 and 10 −6 dilutions ( Fig. 6e,f ). These dose-dependent responses are consistent with behavioural data that ASH are involved in avoidance of higher concentrations of isoamyl alcohol ( Fig. 5b ), but not in attraction to lower concentrations of the odorant ( Supplementary Fig. S2c–e ). These results indicate that ASH sensory neurons are activated by only higher concentrations of isoamyl alcohol and probably induce avoidance behaviour when the odour concentration is higher. Finally, we monitored the responses of AWB sensory neurons ( Fig. 6g,h ). AWB are known to mediate avoidance of the repellent nonanone [12] and it was recently reported that AWB are activated after removal of nonanone [31] . We observed calcium increases in AWB after the removal of isoamyl alcohol, and similar to ASH, maximal responses were observed at 10 −2 dilution, while considerable responses were not detected at 10 −4 and 10 −6 dilutions after the removal of isoamyl alcohol ( Fig. 6h ). These results indicate that AWB sensory neurons are activated by the removal of only higher concentrations of isoamyl alcohol and such high concentration-specific responses may regulate avoidance behaviour. Unexpectedly, calcium increases in AWB were also observed after addition, as well as removal, of 10 −4 dilution of isoamyl alcohol ( Fig. 6g ). There is the possibility that these AWB responses might be related to their functions in attraction to lower concentrations of isoamyl alcohol, because killing AWB caused considerable defects in chemotaxis to it ( Supplementary Fig. S2c,d,f ). Taken together, the pattern and strength of neuronal activities in sensory neurons dramatically change depending on the isoamyl alcohol concentration, and these changes probably regulate the olfactory preference change between lower and higher concentrations of the odorant. Calcium imaging in wild-type animals revealed that each of AWC, AWB and ASH shows odour concentration-dependent responses. We next measured calcium responses of these neurons in the odr-3 mutants, which were defective in odour concentration-dependent behaviour, as shown in Fig. 4a ( Fig. 6i–p ). First, we monitored activities of ASH and AWB neurons in the response to a higher concentration of isoamyl alcohol in the odr-3 mutants, and observed that ASH responses were drastically diminished in the mutants ( Fig. 6m,n ). These results indicate that ODR-3 regulates the olfactory signal–transduction pathway in ASH. AWB calcium responses to isoamyl alcohol in the odr-3 mutants were similar to those in wild-type animals ( Fig. 6o,p ), whereas the defects of isoamyl alcohol avoidance in the odr-3 mutants were rescued by the expression of odr-3 in AWB ( Fig. 4i ). The inconsistency between two experiments might result from the artificial overexpression of odr-3 gene in the rescued line, even though the possibility that ODR-3 functions also in AWB is not completely ruled out. We next monitored AWC ON responses to lower concentrations of isoamyl alcohol in the odr-3 mutants. For the AWC ON calcium responses to isoamyl alcohol, the odr-3 mutants did not show considerable defects compared with wild-type animals at any dilutions tested ( Fig. 6a,b,i–l ). On the other hand, the response of AWC ON to 10 −8 dilution of isoamyl alcohol was considerably impaired in the odr-3 gpa-3 double mutants ( Fig. 6k,l ). These results may be consistent with the behavioural data that the odr-3 gpa-3 double mutants exhibited a severer defect than the odr-3 single mutants in chemotaxis to lower concentrations of isoamyl alcohol ( Fig. 4a ), and suggest that both ODR-3 and GPA-3 mediate signal transduction of lower concentrations of isoamyl alcohol in AWC ON as previously reported [19] . Calcium imaging of sensory neurons in the odr-3 mutants supports our results of cell-specific rescue and knockdown experiments, and suggests that the sensory transduction via ODR-3 in ASH is important for avoidance of higher concentrations of isoamyl alcohol. Although a change of olfactory preference depending on the odorant concentration is empirically known in some organisms including humans ( Fig. 7 ) [1] , [2] , [3] , it is not understood how neural circuits regulate this phenomenon due to the complexity of their neural circuits. In this study, we demonstrated that a variety of attractive odorants become repellants to C. elegans at higher concentrations ( Fig. 1b ). Because C. elegans has simple neural circuits that are fully described, it is an ideal model animal for analysing the mechanisms that regulate how olfactory preference changes depending on the odour concentration. 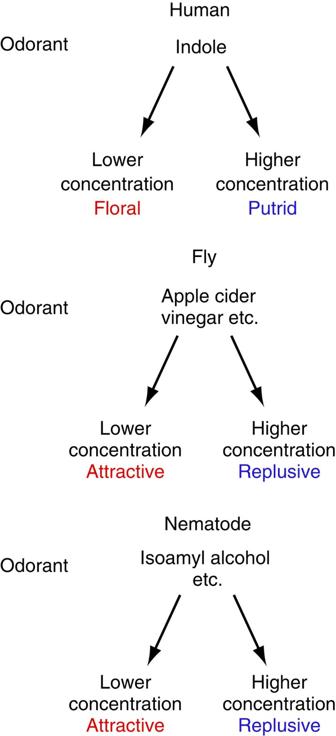Figure 7: Nematode as well as human and fly shows the olfactory preference change depending on odour concentrations. In human, an odorant indole included in jasmines and feces has a pleasant and floral smell at low concentrations, but is putrid when concentrated. InDrosophila, apple cider vinegar induces attraction behaviour at low concentrations, whereas higher concentrations of it cause avoidance. Also inC. elegans, higher concentrations of attractive odorants, which lead attraction behaviour at lower concentrations, induce avoidance behaviour. Figure 7: Nematode as well as human and fly shows the olfactory preference change depending on odour concentrations. In human, an odorant indole included in jasmines and feces has a pleasant and floral smell at low concentrations, but is putrid when concentrated. In Drosophila , apple cider vinegar induces attraction behaviour at low concentrations, whereas higher concentrations of it cause avoidance. Also in C. elegans , higher concentrations of attractive odorants, which lead attraction behaviour at lower concentrations, induce avoidance behaviour. Full size image We also showed that behavioural responses to an odour at different concentrations are mediated by distinct groups of sensory neurons, whose activity patterns dramatically change depending on the odour concentration. AWC sensory neurons were reported to be important for attraction to lower concentrations of odours [8] . On the other hand, our genetic analyses of the odr-3 mutants and laser ablation experiments revealed that ASH sensory neurons have a critical role in avoidance of higher concentrations of isoamyl alcohol. Moreover, calcium imaging showed that AWC neurons respond to the odour only at lower concentrations, whereas ASH neurons respond to only the higher concentration of it. Hence, these results indicate that the information processing of odour concentrations in C. elegans can be primarily explained by the labelled-line theory, where activity in a particular sensory neuron is linked to a specific behavioural output ( Fig. 8 ). This odour concentration-dependent functional segregation of sensory neurons involved in the odour response ensures that animals perform appropriate alternative behaviours such as attraction or repulsion. 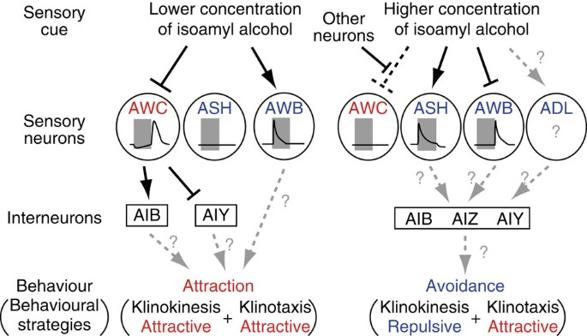Figure 8: A neural network model for chemotaxis to isoamyl alcohol at lower and higher concentrations. It was inferred from previous studies that AWC neurons are activated by removal of isoamyl alcohol at lower concentrations, and regulate AIB interneurons positively and AIY interneurons negatively. Our present study suggests that at higher concentrations, AWB and ASH neurons also show characteristic responses to isoamyl alcohol, whereas AWC fails to respond to it by suppression of other neurons. The attraction behaviour to lower concentrations of isoamyl alcohol is mediated by parallel use of klinokinesis and klinotaxis. Meanwhile, the avoidance of higher concentrations of isoamyl alcohol is mainly regulated by reversed output of the klinokinesis mechanism. Figure 8: A neural network model for chemotaxis to isoamyl alcohol at lower and higher concentrations. It was inferred from previous studies that AWC neurons are activated by removal of isoamyl alcohol at lower concentrations, and regulate AIB interneurons positively and AIY interneurons negatively. Our present study suggests that at higher concentrations, AWB and ASH neurons also show characteristic responses to isoamyl alcohol, whereas AWC fails to respond to it by suppression of other neurons. The attraction behaviour to lower concentrations of isoamyl alcohol is mediated by parallel use of klinokinesis and klinotaxis. Meanwhile, the avoidance of higher concentrations of isoamyl alcohol is mainly regulated by reversed output of the klinokinesis mechanism. Full size image The results of killing AWB sensory neurons and triple ablation including AWB and ASH, compared with ASH single ablation, suggest that AWB have a minor role in the avoidance of higher concentrations of isoamyl alcohol ( Fig. 5b ). Because AWB are known to mediate avoidance of a repulsive odour nonanone and be activated on removal of it [9] , [31] , AWB activation on removal of a higher concentration of (10 −2 diluted) isoamyl alcohol ( Fig. 6h ) would be important for avoidance of it. On the other hand, calcium increases in AWB were observed after addition of 10 −4 diluted isoamyl alcohol ( Fig. 6g ). How is behaviour affected by AWB activation on addition of isoamyl alcohol? We speculate this AWB response may be required for attraction to lower concentrations of isoamyl alcohol, because a slight but statistically significant decrease of attraction to 10 −4 diluted isoamyl alcohol was observed in animals lacking AWB functions ( Supplementary Fig. S2d ). Taken together, AWB might regulate both attraction and avoidance behaviour depending on the odour concentration ( Fig. 8 ). It has also been reported that a single olfactory neuron can switch from attraction to repulsion towards lower concentrations of an attractive odorant [32] . Hence, a mechanism different from the labelled-line theory might also contribute to the regulation of the olfactory preference switch depending on the odour concentration. Recently, researchers described a neuronal mechanism underlying the olfactory behavioural switch depending on the odour concentration in Drosophila [33] . Apple cider vinegar, a food odour, at a low concentration triggers robust attraction by exciting several glomeruli that mediate attraction. At higher concentrations, vinegar activates a glomerulus that mediates avoidance in addition to activating the glomeruli that elicit attraction. In contrast, in C. elegans , a higher concentration of isoamyl alcohol fails to evoke the response in the AWC ON sensory neuron, which mediates attraction at lower concentrations of the odorant. This suppression of activity of the sensory neuron that is important for attraction, under a higher concentration of attractive odorant, could be a reasonable mechanism for the efficient preference switch depending on the odour concentration in C. elegans . Worm culture and strains C. elegans strains were cultured at 20 °C using a standard technique [34] on NGM plates with Escherichia coli NA22 as a food source unless otherwise indicated. Strains used were all derivatives of C. elegans var. Bristol: wild-type N2, CX2205: odr-3(n2150) , NL332: gpa-1(pk15) , NL334: gpa-2(pk16) , NL335: gpa-3(pk35) , NL1137: gpa-5(pk376) , NL1146: gpa-6(pk480) , NL787: gpa-11(pk349) , NL2330: gpa-13(pk1270) , NL797: gpa-15(pk477) , MT4866: let-60(n2021) , JN130: let-60(n1046) , CX10: osm-9(ky10) , NM1380: egl-30(js126) , JN372b: gpc-1(pe372) , JN5: goa-1(n1134 ), JN727: tax-2(p691) , JN730: tax-4(p678) and MT7929: unc-13(e51) . Behavioural assays Population chemotaxis assays were performed with modified assay plates shown in Fig. 1a (ref. 8 ). One μl each of 10 −2 diluted odorant or 1, 5 or 10 μl each of undiluted odorant was spotted on two points (plus marks) at one end of the assay plates, and 1 μl of 1 M sodium azide was spotted on two points at both ends of the plates. Animals were placed on the centre of the plate. After 1 h, the number of animals in each area of the plate (N+ and N−) was counted and the chemotaxis index was calculated. Chemotaxis index=[(N+)−(N−)]/[(N+)+(N−)]. Odour adaptation (olfactory plasticity) assays were performed as previously described [35] . Animals were soaked in a buffer without (mock-conditioned) or with (conditioned) isoamyl alcohol at 10 −4 dilution for 1 h and then tested for chemotaxis to same odorant at 10 −2 dilution. Single-animal chemotaxis assays were performed using modified assay plates, shown in Fig. 5a (ref. 9 ). Because it is difficult to prepare a lot of cell-ablated animals, we quantified the behaviours of individual animals by manually recording their tracks. The single-worm chemotaxis index was calculated as shown in Fig. 5a . Animals used for single animal assays were cultured with E. coli OP50 as a food source. Cell-specific knockdown of odr-3 function The construction of transgenes to knockdown functions of a targeted gene in a specific neuron was performed as follows [36] . The targeted gene ( odr-3 ) and the chosen cell-specific promoter were amplified separately, and then the two amplified fragments were fused in a second PCR. The targeted odr-3 region (2.3-kb genomic sequences) was amplified with two primers Tf=5′-AATTCTTCATAGCAACGGATTC-3′ and Tr=5′-CTGATTAGTGTCTGTAGCGC-3′. As cell-specific promoters, sra-6 and str-1 promoters were used to express the targeted gene in ASH and AWB neurons, respectively. To yield sense and antisense constructs, a part of sequences of Tf or Tr primer was added to sequences of the reverse primer used for the amplification of the chosen cell-specific promoter. The two products were mixed and injected with a visible selectable marker in wild-type animals. Laser ablation Laser ablation was performed using Micropoint equipped with Zeiss upright microscope Axioscope at the L1–L4 stage depending on the neuron [37] . Killed neurons were identified by either DiO filling (for ADL and ASH) or using fluorescence of green fluorescent protein or Venus expressed in the target cells. Mock-ablated animals were used as a control of each experiment. Fluorescent lines used were Is[npr-9p :: Venus] for AIB, Ex[ttx-3p :: GFP] for AIY, Ex[lin-11p :: nlsGFP] for AIZ, Ex[nmr-1p :: nlsGFP] for AVA and AVE, Ex[odr-10p :: Venus] for AWA, Ex[str-1p :: GFP] for AWB and Ex[gcy-10p :: GFP] for AWC. Multiworm tracking system We used a camera (Lw575M-IO; ARGO) and a LED illumination (HPR-150SW; CCS) equipped with a digital power source (PD2-3024; CCS). Images of 50–150 animals on an individual assay plate were captured. The interval between image captures was 500 ms, and the recording time was 1 h. Saved images were analysed using custom software based on Lucam Capture (ARGO) and OpenCV, by which each image was binarized by thresholding after background subtraction and the centroids of the animals were extracted. The design of the plate shown in Fig. 1a was used unless otherwise indicated. The klinotaxis data in Fig. 3f was obtained by using the plate design shown in Fig. 3e . Sodium azide was not spotted on the plate. Analysis of tracking data Two centroids of the objects, which are the closest between two images, were connected, and defined as one track. If more than two animals overlapped on the plate, the object is not recognized as an animal and the tracks are terminated at that point. The tracks shorter than 1 mm were removed from tracking data. The existence frequency of animals was calculated by using the formula (the total sojourn time of animals existing in a region at some distance from an odour source)/(the total sojourn time of animals existing in the whole region on an agar plate). The distance from odour source (64 mm maximum) was divided into 2 mm bins. The assay time (3,600 s total) was divided into 150 s bins. A sharp turn was defined as >100° change of the direction of locomotion, and consecutive sharp turns separated by <3.18 s were defined as a pirouette. On the basis of these criteria, locomotion was separated into pirouettes and the rest of the tracks, which were called runs. Pirouettes and the run parts were used to quantify klinokinesis and klinotaxis, respectively. Bearing ( θ ) and curving rate were determined as shown in Supplementary Fig. S1a . All angles were defined as positive for clockwise rotation. Calculation of the pirouette index, the basal pirouette frequency and the weathervane index was performed as previously described [5] with some modifications. During klinokinesis, worms respond to chemical gradient tangential to the direction of locomotion [6] ( Fig. 3a ). On the other hand, during klinotaxis, worms respond to the chemical gradient perpendicular to the direction of locomotion [5] ( Fig. 3b ). Therefore, the cosine θ and the sine θ were used to quantify klinokinesis and klinotaxis, respectively. In analyses of klinokinesis, the relationship between the cosine θ and the probability of a pirouette was calculated ( Supplementary Fig. S1b ). All data points of tracking data were classified into 10 groups according to the cosine θ , and the average was plotted for the midpoint of cosine θ in each rank. The pirouette index was defined as the negative slope of the regression line. The y-intercept of this regression line is a measure of the basal pirouette frequency. Averaged pirouette index and basal pirouette frequency per assay were presented. In analyses of klinotaxis, the relationship between the sine θ and average curving rate was calculated ( Supplementary Fig. S1c ). All data points of tracking data were classified into 10 groups according to sine θ . The weathervane index was defined as the slope of the regression line. Averaged weathervane index per assay was used for further analyses. Algorithm of computer simulation The simulator renewed the position and direction of movement of a model animal every 500 ms. Movement of the animal was modelled by a correlated random walk model, with the velocity of the model animal set to a constant value of 0.22 mm s −1 , which is the average velocity of wild-type animals in gradient of a higher concentration of isoamyl alcohol. The curving rate (change of movement direction per unit length of progression, ° mm −1 ) of the animal followed a first-order autoregression, namely, where k =0.933 is a decay constant determined from the measurement of decay rate shown as Supplementary Fig. S2A in the previous paper [5] , and ξ i N (0,11.6) is a Gaussian white noise whose standard deviation was determined also from real measurements [5] . When klinotaxis was implemented, the curving bias was added as follows, where ψ i is actual curving rate, θ is the bearing of the odour source and α is the weathervane index whose values are shown in Fig. 3h . A pirouette occurred at the probability based on the basal pirouette index in Supplementary Fig. S1d . After a pirouette occurred, new θ was set by adding a delta θ -value randomly selected from the distribution in Supplementary Fig. S1e . When klinokinesis was incorporated, a pirouette occurred at the probability based on the pirouette index in Fig. 3g . Calcium imaging and statistics Animals used for calcium imaging were cultured with E. coli OP50 as a food source. CX6632: Ex[sra-6p :: GCaMP] (a kind gift from C. Bargmann) was used for ASH imaging. GCaMP2 was expressed in AWC ON and AWB by str-2 and str-1 promoter, respectively. An animal expressing GCaMP was fixed in a microfluidic device [27] . Before recordings, nose tips of the worms were washed with imaging buffer (5 mM potassium phosphate (pH 6.0), 1 mM CaCl 2 , 1 mM MgSO 4 , 350 mOsm glycerol) for 5 min. An odour was administered for 72 s before removal. We measured GCaMP calcium responses on addition and removal of odour in the same animals. The fluorescent images were captured using Leica invert microscope (DMI6000 B) with ×63 oil immersion objective lens and ImagEM CCD camera (Hamamatsu photonics). Images were collected every 800 ms with an exposure time of 500 ms. The region of interest (ROI) was defined by highlighting the desired cell body in the animal [13] . A data log file was created for each stack with the background-subtracted fluorescence intensity of ROI, and was used for subsequent analyses. The fluorescence intensity in a 10-s period (time=1–10 s) was averaged and defined as F0. The percent change in fluorescence value of ROI relative to F0 was plotted for all stacks. For statistical analyses, the averaged fluorescence value was calculated for each animal in the 10 s before and after shifts from the buffer to the buffer containing an odour or from the buffer containing an odour to the buffer. Genetic ablation and cloning of Mouse Caspase 1 Mouse Caspase 1 (mCasp1) cDNA (1,209 bp) was amplified by PCR from cDNA library of C57BL/6 mouse, and then inserted into the pPD-DEST vector with Gateway system (Invitrogen). Genetically cell-ablated lines used in this study were Is[ceh-36p::mCasp1] for AWC, Is[sra-6p :: mCasp1] for ASH and Is[str-1p :: mCasp1] for AWB. How to cite this article: Yoshida, K. et al . Odour concentration-dependent olfactory preference change in C. elegans . Nat. Commun. 3:739 doi: 10.1038/ncomms1750 (2012).